Cumulative human impacts on marine predators Stressors associated with human activities interact in complex ways to affect marine ecosystems, yet we lack spatially explicit assessments of cumulative impacts on ecologically and economically key components such as marine predators. Here we develop a metric of cumulative utilization and impact (CUI) on marine predators by combining electronic tracking data of eight protected predator species ( n =685 individuals) in the California Current Ecosystem with data on 24 anthropogenic stressors. We show significant variation in CUI with some of the highest impacts within US National Marine Sanctuaries. High variation in underlying species and cumulative impact distributions means that neither alone is sufficient for effective spatial management. Instead, comprehensive management approaches accounting for both cumulative human impacts and trade-offs among multiple stressors must be applied in planning the use of marine resources. Marine predators provide resilience and health to marine ecosystems [1] . Changes in the abundance and distribution of marine predators can result in alterations in the structure and function of ecosystems through trophic cascades and effects on ecosystem processes such as carbon sequestration and the increased spread of disease [2] , [3] . These changes in marine predator abundance and distribution can also compound human impacts by, for example, increasing an ecosystem’s susceptibility to invasive species or loss of biodiversity [4] , [5] . Further, protecting the large and varied habitat of marine predators can indirectly protect other species or the larger ecosystem. Predators can serve as indicators of ecosystem health [6] , [7] as marine predators are critical components of marine ecosystems, they have been identified as a key element of spatial and ecosystem-based management, such as marine protected area design and systematic conservation planning [8] , [9] . Fundamental to spatial and ecosystem management approaches is an understanding of both the distribution of predators and the spatially explicit cumulative impacts of multiple stressors on species groups [10] , [11] , [12] , [13] . Many pelagic marine predators traverse thousands of kilometres in a year, linking disparate ecosystems and crossing international boundaries [14] , [15] , [16] , yet often concentrate within small-scale ‘hotspots’ to breed or forage [17] , [18] . The California Current System (CCS) contains many hotspots used by predator species from across the Pacific Ocean because of its predictable nutrient input from coastal upwelling [19] , [20] . In the CCS the location and intensity of certain drivers (that is, human activities such as fishing) or stressors (that is, the means by which human activities have effects, such as fishing pressure) are well known, and in some cases so are the specific impacts (that is, resulting consequences of stressors on species). However, cumulative human impacts on predators in this hotspot are unknown and effective ecosystem-based management including predators requires such information. Marine predators are often exposed to varying levels of multiple anthropogenic stressors because of their long distance movements [15] , [21] . Determining cumulative risk to their populations is therefore challenging but critical, given that cumulative impacts may represent synergistic effects that exceed the effect of individual stressors [22] . The potential impacts of anthropogenic stressors on predators has been examined with respect to population dynamics, critical life stages or the simple spatial overlap of predators and stressors [11] , [13] , [15] , [23] , [24] . Most studies, however, investigate only a single impact or stressor, a single species or incorporate only the presence/absence of predators rather than a more quantitative habitat assessment to integrate relative habitat use and the potential impacts of human activities and their associated stressors [11] , [15] , [23] , [24] . This piecemeal approach to determining cumulative risk to marine predator populations can be ineffective and ecologically misleading because cumulative impacts are not considered and the effects of transferring human activities to different regions in the process of mitigation are overlooked. Assessments that look across the habitat use of multiple species and incorporate cumulative impacts across stressors will be the most advantageous to managers considering trade-offs among strategies and looking to plan management over large spatial and temporal scales [10] , [25] . Spatially explicit analyses of anthropogenic impacts on predators must also be coupled with analyses that assess whether current spatial management measures are effectively protecting habitat, such that they likely reduce cumulative impacts to marine predators. Five National Marine Sanctuaries (hereafter ‘sanctuaries’) occur along the US West Coast and are the largest marine protected areas in the region, covering over 38,000 km 2 of the US West Coast exclusive economic zone (EEZ). The sanctuaries were created with the ‘purpose of preserving or restoring (marine) areas for their conservation, recreational, ecological or aesthetic values’ [26] . The sanctuaries are important habitat and a potential protection mechanism for marine predators [11] , but an assessment of how well the sanctuaries reduce overall (that is, cumulative) impacts on marine predators has never been conducted. Advancing our understanding of marine predators and anthropogenic impacts on them requires assessments that look across a suite of species and their relative habitat use, incorporate cumulative impacts of multiple stressors and assess the relative sensitivity of species to different potential stressors, all within a spatial context. In this study, we use satellite- and light-based geolocation tracking data from the Tagging of Pacific Predators project to determine the distribution and key habitats of eight protected predator species across three taxa groups within the US waters of the CCS. We then determine the relative impact of 24 spatially explicit and quantified anthropogenic stressors on individual marine predator species in the US EEZ to create a novel metric (cumulative utilization and impact, CUI). This metric identifies overlap between species and impacts and identifies where potential impacts on those species are greatest. We use a suite of key predator species that span a variety of ecological roles and life histories (that is, central place foragers, capital breeders and migratory breeders) to determine their distribution and potential risks to them in the US West Coast EEZ, including in relation to the sanctuaries. We address several questions relevant to management of the CCS, including: what are the distributions of key species groups and relevant human impacts in the CCS? Are there differences in the patterns of distribution across species groups? What are the cumulative impacts on marine predators in the CCS? Are current management measures, particularly the National Marine Sanctuary system, encompassing key areas for marine predators? And where are spatial mitigation efforts likely to have the greatest effects? We find some of the highest CUI regions on the continental shelf and in the sanctuaries, but suggest means of mitigating impacts and paths forward to better management of marine predators. Animal distribution All of our species groups are widely distributed across the US West Coast EEZ; however, utilization distributions (UDs) that is, the probability of an animal being found in a given cell [27] ) showed that areas of high use are regionally concentrated ( Fig. 1 ). 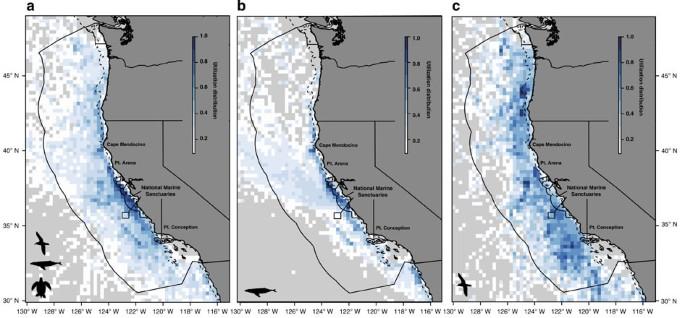Figure 1: Species group UDs. UDs (the probability of an animal being found in a given cell27) of (a) all species combined (n=685), (b) marine mammals (n=384) and (c) seabirds (n=283) in the California Current based on tracking data. Outer solid line represents the US EEZ; solid inner lines represent the US National Marine Sanctuaries; hashed lines represent the 200-m depth contour. The mean UD of all species combined is greater on the continental shelf (Welch’s t -test, t 281 =11.0, P <0.001) with 76.7% of core UD area on the shelf ( Table 1 ; Fig. 1 ). Mean seabird UDs are greater on the continental shelf (Welch’s t -test, t 281 =15.8, P <0.001) but they use large areas of the offshore EEZ with 80.4% of core UD areas found off shelf ( Table 1 ; Fig. 1 ). Similarly, marine mammal and leatherback sea turtle mean UDs are greater on the shelf (Welch’s t -tests; marine mammals, t 251 =7.81, P <0.001; sea turtles, t 74 =4.58, P <0.001), although they are not as widespread, and core areas are concentrated more nearshore compared with seabirds ( Table 1 ; Fig. 1 ). There is a significant difference detected among species groups both on and off the continental shelf (one-factor analysis of variance (ANOVA); on shelf: F 2,511 =18.26, P <0.001; off shelf: F 2,2554 =181.86, P <0.001; Table 1 ). Post hoc comparisons using Tukey’s honestly significant difference (HSD) test indicated that the mean UD of seabirds is greater than marine mammals and leatherback sea turtles, both on and off the shelf ( P <0.001), and that the marine mammal mean UD is greater than turtles on the shelf ( P <0.001; Table 1 ). Mean UDs are greater in the sanctuaries for all species combined (Welch’s t -test, t 62 =7.96, P <0.001) compared with outside the sanctuaries and marine mammals (Welch’s t -test, t 41 =4.47, P <0.001) with the majority of core UDs found in the sanctuaries for these groups (57.0 and 68.5%). However, for seabirds (Welch’s t -test, t 64 =−1.60, P =0.114) and leatherback sea turtles (Welch’s t -test, t 19 =2.52, P =0.021) there is no difference, although 28.3% and 70.4%, respectively, of their core areas are detected in the sanctuaries. Post hoc comparisons indicate that the mean marine mammal UD is greater than the mean seabird UD within the sanctuaries (one-factor ANOVA; in sanctuaries: F 2,88 =8.67, P <0.001), whereas the mean seabird UD is greater than leatherback sea turtles outside the sanctuaries (one-factor ANOVA; outside sanctuaries: F 2,395 =6.20, P <0.001; Table 1 ). Figure 1: Species group UDs. UDs (the probability of an animal being found in a given cell [27] ) of ( a ) all species combined ( n =685), ( b ) marine mammals ( n =384) and ( c ) seabirds ( n =283) in the California Current based on tracking data. Outer solid line represents the US EEZ; solid inner lines represent the US National Marine Sanctuaries; hashed lines represent the 200-m depth contour. Full size image Table 1 Continental shelf and NMS influence. Full size table Cumulative impacts distribution Cumulative impacts of anthropogenic activities (that is, underlying human stressors weighted by species vulnerability but without species distributions incorporated) vary considerably among species groups ( Fig. 2 ). Cumulative impacts encompass the entire EEZ ( Fig. 3 ) but they have higher values nearshore and within the sanctuaries for all species groups. High values are also found offshore of Northern California for both seabirds and leatherback sea turtles driven largely by fishing, pollution and climate impacts. The mean cumulative impact is greater on the shelf than off for all groups (Welch’s t -tests; all species, t 298 =17.29, P <0.001; marine mammals, t 295 =17.37, P <0.001; seabirds, t 297 =20.18, P >0.001; leatherback sea turtles, t 309 =15.49, P <0.001), with greater than 90% of the core area of all cumulative impacts found on the shelf across species groups ( Table 1 ). Post hoc comparisons using Tukey’s HSD tests indicate the mean cumulative impact value on leatherback sea turtles is lower than both seabirds and marine mammals on the shelf (one-factor ANOVA; F 2,861 =4.11, P =0.018). Off the shelf, cumulative impact on marine mammals is greater than that on either seabirds or sea turtles, and the impacts on sea turtles are greater than that on seabirds (one-factor ANOVA; F 2,3309 =200.25, P >0.001). Within-group comparisons indicate that the mean cumulative impact is also greater within the sanctuaries for all groups (Welch’s t -tests; all species, t 113 =5.36, P <0.001; marine mammals, t 112 =4.74, P <0.001; seabirds, t 114 =5.97, P >0.001; leatherback sea turtles, t 113 =5.27, P <0.001), with greater than 30% of all core cumulative impact cells found within the sanctuary boundaries ( Table 1 ). No differences are found among species groups within the sanctuaries (one-factor ANOVA; F 2,312 =0.50, P =0.610); however, post hoc comparisons indicate impacts are greatest outside the sanctuaries for marine mammals, followed by leatherback sea turtles, and then seabirds (one-factor ANOVA; F 2,3858 =36.08, P <0.001). 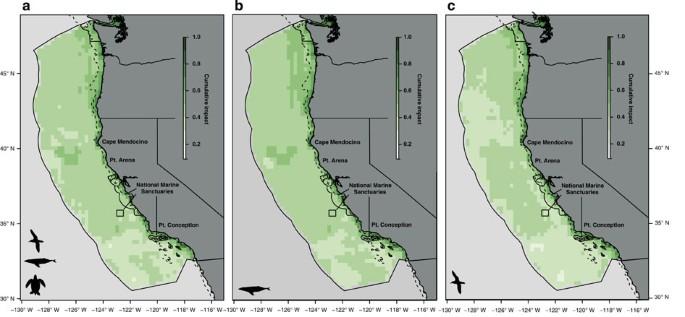Figure 2: Cumulative impact distribution. Distribution of cumulative impacts (that is, stressor data weighted by species vulnerability but without animal distributions included;n=24 impacts) in the US EEZ for (a) all species combined, (b) marine mammals and (c) seabirds. Outer solid line represents the US EEZ; solid inner lines represent the US National Marine Sanctuaries; hashed lines represent the 200-m depth contour. Figure 2: Cumulative impact distribution. Distribution of cumulative impacts (that is, stressor data weighted by species vulnerability but without animal distributions included; n =24 impacts) in the US EEZ for ( a ) all species combined, ( b ) marine mammals and ( c ) seabirds. Outer solid line represents the US EEZ; solid inner lines represent the US National Marine Sanctuaries; hashed lines represent the 200-m depth contour. 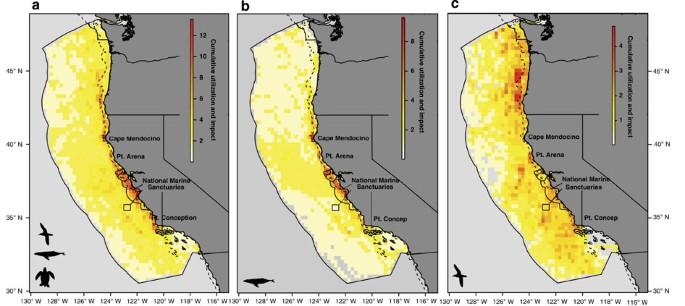Figure 3: CUI distribution. CUI that combines tracking data and cumulative impact data for marine predators in the US EEZ for (a) all species combined, (b) marine mammals and (c) seabirds. Outer solid line represents the US EEZ; solid inner lines represent the US National Marine Sanctuaries; hashed lines represent the 200-m depth contour. Full size image Figure 3: CUI distribution. CUI that combines tracking data and cumulative impact data for marine predators in the US EEZ for ( a ) all species combined, ( b ) marine mammals and ( c ) seabirds. Outer solid line represents the US EEZ; solid inner lines represent the US National Marine Sanctuaries; hashed lines represent the 200-m depth contour. Full size image CUI distribution The highest CUI, (for example, the integration of UDs and cumulative impacts) values are found within the sanctuaries and close to the coastal region between Point Arena south to Monterey Bay for all species and for marine mammals and leatherback sea turtles, whereas high seabird CUI values are found further north, particularly along the shelf break off the coast of Oregon ( Fig. 3 ). Mean CUI is greater on the shelf for all species groups (Welch’s t -tests; all species, t 270 =8.35, P <0.001; marine mammals, t 243 =7.64, P <0.001; seabirds, t 285 =11.32, P <0.001; leatherback sea turtles, t 75 =3.82, P <0.001), and nearly 100% of core CUI cells are found on the shelf for all species and for marine mammals and sea turtles, whereas for seabirds 82.1% of core cells are on shelf. Post hoc comparisons indicate differences among all species both on (one-factor ANOVA; F 2,511 =33.70, P <0.001) and off the shelf (one-factor ANOVA; F 2,2554 =189.14, P <0.001), although direction of the differences varies. On the shelf, mean CUI for marine mammals is greater than that for either seabirds or sea turtles ( P <0.001), whereas off the shelf, mean CUI for seabirds is greater than the other two groups ( P <0.001). In addition, mean CUI is greater in the sanctuaries for all groups (Welch’s t -tests; all species, t 107 =7.52, P <0.001; marine mammals, t 243 =7.64, P <0.001; seabirds, t 285 =11.32, P <0.001; sea turtles, t 75 =3.82, P <0.001), and greater than 80% of core CUI cells are found in the sanctuaries for all species combined and for marine mammals and sea turtles, whereas for seabirds only 23.9% of core cells are found in the sanctuaries. Post hoc comparisons indicate that CUI is greatest both inside and outside the sanctuaries first for marine mammals, followed by seabirds, and then sea turtles (inside sanctuaries: one-factor ANOVA; F 2,253 =21.54, P <0.001; outside sanctuaries: F 2,2812 =172.14, P <0.001; Table 1 ). Influence of CUI layers Climate CUI layers (ocean acidification, ultraviolet radiance anomalies and sea surface temperature anomalies) have greatest contributions to the overall CUI value (for example, high R 2 -values or spatial correlations between individual CUI layer and overall CUI, Supplementary Table S1 ), probably because of the widespread nature of these stressors, although the combined CUI values from climate CUIs are stronger inshore ( Supplementary Fig. S1 ). The contribution of fishing CUIs to the overall CUI value shows variable distribution among species groups, with higher fishing CUI values along the shelf break for seabirds and greater offshore for marine mammals, but with the greatest CUI values for fishing occurring within the sanctuaries for all species combined ( Supplementary Fig. S2 ). Pollution CUI layers (ocean and coastal pollution, organic and inorganic pollution and ocean deposition) influences the overall CUI across groups and are stronger inshore for all species because these stressors primarily occur in coastal areas; the region with the highest CUI values for pollution for all species combined occurs around Monterey Bay within the sanctuaries, as well as near Cape Mendocino ( Supplementary Fig. S3 ). Both shipping and CUI layers that result in direct impact on marine predators are greater on the continental shelf compared with pelagic regions for both marine mammals and seabirds ( Supplementary Figs S4 and S5 ). CUI layers with direct impacts on marine predators, particularly for marine mammals, are distributed largely on the continental shelf and within the sanctuaries. Some coastal CUI layers, such as human use via beach access and coastal engineering, also indicate strong potential impacts on marine mammal species because of the proximity of some of these species to the coasts during both breeding and foraging stages ( Supplementary Tables S1 and S2 ; Supplementary Fig. S6 ). These results should be interpreted with caution, however, because the underlying stressor occurs only near the coast. Although some marine mammals come in contact with shorelines, others may never be under direct impact of coastal stressors such as human use of beaches. Despite not having a large influence on the overall CUI, a number of other CUI layers, such as coastal waste, shipping and high-bycatch demersal fisheries, have moderate potential impacts in specific, localized areas on all species groups, as indicated by the high maximum values and large s.d. of the individual pixels. Ocean pollution and low-bycatch demersal fishery CUI layers are highly correlated with the overall CUI and have strong localized effects on seabirds. Leatherback sea turtle CUI patterns are more highly correlated with ocean pollution and shipping than is the case for other species, although climate CUI layers are similarly important across all species. This is the first attempt to create a spatially explicit understanding of potential cumulative impacts of human activities on marine predators. We combine tracking data for a broad suite of marine predators with human stressor data weighted to reflect expected impacts specific to those species. The CUI metric is novel in its combination of both relative habitat uses across a broad suite of marine predators and spatial impacts specific to each species. We use the CUI to determine where important species habitat and high-risk areas are likely to coincide within the CCS. The heterogeneous patterns across marine predator habitat (that is, UDs), cumulative impacts (that is, underlying human stressors weighted by species vulnerability but without species distributions incorporated) and CUI (that is, combined UD and cumulative impacts) indicate that there is substantial variability in how animals and anthropogenic impacts are distributed. This highlights the need to understand the potential cumulative impact of the full suite of stressors on multiple species, and understand how these impacts vary among species to design and implement effective and efficient management strategies. Although marine predators are distributed across the expanse of the US EEZ (and beyond), their distributions are concentrated in specific regions. All species are more concentrated along the continental shelf (76.7% of core UD cells on the shelf) but these patterns varied significantly among species groups ( Fig. 1 ), largely because of differences in the life histories and trophic levels of the species [14] , [16] , [18] , [28] , [29] , [30] , [31] , [32] . Cells with high CUI values are also distributed close to or on the continental shelf, with a large proportion within sanctuary boundaries (82.6% of core CUI cells in the sanctuaries) across all species ( Fig. 3 ). A number of areas have high CUI values, particularly the central coast of California for marine mammals and leatherback sea turtles, and off the coast of central Oregon for seabirds. Prominent headlands such as Point Arena, Cape Mendocino and Point Conception are areas of high CUI for marine mammals and seabirds because of the increased abundance of predators associated with upwelling-driven productivity found in these regions, as well as the proximity to the coastline and associated human impacts [17] , [20] . Cumulative impacts are also distributed closer inshore than offshore for all species groups, and the majority of core cumulative impact cells are found on the continental shelf (>90% for all groups), with a high percentage also found within the sanctuary boundaries (>30% for all groups; Table 1 ). These results are not particularly surprising as most human stressors concentrate near human population centres [12] . Interestingly, however, all species groups—and particularly seabirds—have more core CUI cells and, in some cases, more cumulative impact core cells on the shelf and in the sanctuaries despite having a more core UD cells offshore and outside of the sanctuaries, indicating that impact and animal distributions cannot be decoupled. Knowledge of both the distribution of marine predators and impacts using a single quantified metric such as the CUI is therefore important to understand where management efforts could be best directed. Impacts vary in their intensity and in how they affected species ( Supplementary Figs S1–S6 ; Supplementary Table S2 ; Supplementary Note 1 ). Climate stressors have the greatest potential impacts on all species combined, but marine mammals, many of which breed in the CCS [18] , [33] , [34] , are potentially more sensitive to coastal stressors than other species groups, whereas seabirds and leatherback sea turtles are likely more sensitive to fishing and pollution than the other species groups ( Supplementary Table S2 ). Given variable vulnerability among species, our approach can be used to determine where sensitive areas occur, and also when and where potentially harmful human activities can be safely conducted, reducing the areas where management and restrictions need to be implemented. This understanding is critical for effective systematic conservation planning processes, particularly those that explicitly consider human uses of marine systems, as it can be used as a first step to put ecological and economic trade-offs in a spatial context [9] . High spatial correlation between individual CUI layers (for example, ultraviolet radiation, fishing and so on) and the overall CUI score, as indicated by high R 2 -values, indicates the influence of individual CUI layers on the overall CUI patterns ( Supplementary Table S1 ). Per-pixel contributions to CUI scores indicate localized impacts of individual CUI layers. Spatial correlations and per-pixel contributions therefore provide insight into which stressors are widespread and require large-scale, multifaceted mitigation versus those that are localized and can be mitigated using regional approaches. For example, fishing CUI layers are distributed unevenly across the US EEZ as indicated by low spatial correlations with the overall CUI score but fishing has high maximum pixel values relative to other impacts indicating potential high localized impacts ( Supplementary Table S1 ; Supplementary Fig. S2 ). Fishing impacts may be mitigated using techniques such as time-area closures, bycatch reduction devices and modification of fishing methods [35] . By contrast, climate CUI layers are widespread as indicated by high spatial correlations with the overall CUI score and moderate maximum pixel values ( Supplementary Table S1 ; Supplementary Fig. S1 ). Reduction of climate stressors will require global-scale effort and international cooperation. Mitigation of the impacts from these stressors might occur locally, however, through protection of microrefugia habitats or prey resources, or adaptive management practices [36] , [37] . Still, the empirical impacts of multiple stressors on individuals and populations of marine predators require additional study. Impacts may not be simply additive, as assumed in this study, but rather synergistic or antagonistic as has been found for ecosystems [22] . Field studies that measure different combinations of stressors and their resulting individual and population-level impacts are critical to designing effective management strategies. We can make direct comparisons of how impacts differ among ecosystems and predators by comparing species-specific results presented here to previously published ecosystem-scale cumulative impacts within the same region using the same stressor data [38] . A number of climate layers, including change in the sea surface temperature anomalies and ultraviolet radiation, and pollution variables such as ocean-based pollution, have a strong influence on the overall CUI for predators and on overall cumulative impact maps for ecosystems [38] . This suggests that mitigation for some stressors will have impacts across multiple ecosystem components. The influence of other layers, such as those related to fishing, vary across species and were markedly different than ecosystems, highlighting that some mitigation strategies will need to be tailored to specific species or ecosystems. The sanctuaries are key regions of both predator distribution and high CUI for most species, even with the removal of CUI layers that have only indirect impacts on marine predators ( Table 1 ; Supplementary Fig. S5 ). Although ecosystem-level protection including protection of predators was part of the intent in the National Marine Sanctuaries Act, the protective capacity of the sanctuaries are limited [39] . Sanctuaries on the US West Coast have largely been designed to reduce impacts from oil and gas exploration and promote marine research; they lack a mandate for specific protections for marine predators [39] . Despite this potential limitation, key areas for marine predators already fall within the footprint of the sanctuaries, affording the opportunity to better protect marine predators through legislative changes that could increase the sanctuary’s protective capacity. This could be achieved by restricting potentially harmful activities within and near the sanctuaries when marine predators are present in large numbers. Increased monitoring of human exploitation and predators within sanctuaries could also aid reducing cumulative impacts on predators, particularly when used in concert with decision support systems such as integrated ecosystem assessments [25] . Existing management strategies that focus on individual species and individual risks can inform more holistic approaches to ensure that shifts in effort are not having unforeseen negative consequences. Risk assessments need to consider cumulative impacts, human uses of marine ecosystems and environmental variability with explicit attention to iteratively evaluating management strategies and the trade-offs between ecological and socioeconomic objectives. Our findings highlight the need to consider the legislative capacity to mitigate stressors across agencies, sectors and governments, and integrated ecosystem assessments offer a potentially strong tool to do so. In addition, systematic conservation planning is inherently based on spatial management (although non-spatial management measures may be considered in the process), includes iterative feedbacks, and has a proven history of success [9] , [40] . Inclusion of cumulative impacts and biological data in a spatial context, such as described here, are important components of such processes that may lead to more effective management practices. Here we use the distribution of individuals from eight species across three guilds, but this approach could readily be applied to other species, as well as in other marine ecosystems. Given that we examined a subset of populations, additional effort could find other important areas for these species and this approach could ultimately be expanded to incorporate population-level dynamics. Further examination of species that represent additional ecological niches, additional life stages (for example, juveniles) and other sectors of the population will increase the robustness of the results from this approach [41] . Long-term tracking data sets may help discern the stability of patterns over time and integration with new biological monitoring techniques (for example, glider surveys) may help clarify the underlying oceanographic and biological resources that are driving the high potential impact regions. It is also important to recognize that many marine predators are highly mobile in both space and time, and stationary protection (for example, marine protected areas) will only afford protection to portions of populations for only small windows of their life history [42] , [43] . Dynamic spatiotemporal management measures based on predator distribution and known human activities would maximize areas open to human use while minimizing harmful impacts and needs for enforcement [44] , [45] . Cumulative impacts on predators within the US EEZ may also be confounded at the population level by impacts at distant breeding or developmental areas [46] . Some of the most serious stressors are themselves not static (that is, climate change) [47] . As the ocean warms, the distribution of animals and marine resource exploitation by humans will further change. Predictive models of these evolving distributions validated with ongoing tracking and monitoring studies will be critical for fine tuning the implementation of management and conservation measures through the 21st century [37] . Movement patterns of marine species also provide opportunities for human activities to occur at different times with reduced risk to predators, for example, during seasons when some predators depart the CCS for distant foraging grounds [19] , [48] . Understanding the dynamic nature of predators and human activities in both space and time can allow for the development of more precise and effective management, reducing impacts on both species and the humans that rely on ocean ecosystems in domestic and international waters [40] , [44] , [45] , [49] . A number of management bodies have already articulated the need to access and understand cumulative impacts within marine systems [50] , [51] . Marine predators are critical components of marine ecosystems, and impacts on their populations can resonate throughout the larger ecosystem through trophic cascades [2] . Regions of high potential impact on predators are concentrated on the continental shelf and within the sanctuaries. The distribution of potentially harmful impacts, however, is related to important human activities that yield both social and economic benefits (for example, tourism and fishing) that cannot be simply halted to prevent ecosystem disturbance. Thus, cumulative impacts to marine predators have the potential to reverberate across both socioeconomic and ecological systems. Our results show that we have the data and monitoring ability to develop strategies to effectively mitigate impacts and manage species simultaneously. This could aid in management approaches that more effectively balance human and ecological needs. Animal tracking We used 685 individual tracks spanning over 5 years (June 2003–January 2009, Fig. 1 ; Supplementary Table S3 ) from eight species of marine predators in three species guilds: marine mammals (blue whales ( Balaenoptera musculus ), humpback whales ( Megaptera novaeangliae ), California sea lions ( Zalophus californianus ), northern elephant seals ( Mirounga angustirostris )), pelagic seabirds ((black-footed albatrosses ( Phoebastria nigripes ), Laysan albatrosses ( Phoebastria immutabilis ), sooty shearwaters ( Puffinus griseus )), and the only sea turtle species that spans a large portion of the California Current in US waters, the leatherback sea turtle ( Dermochelys coriacea ; Supplementary Table S3 ). The purpose of this exercise is not to look at species impacts at a population level but rather to use a multispecies approach to understand human impacts on marine predators on the scale of the CCS; hence, we consider individuals from known important rookeries or feeding grounds. All of these species are protected by US law under the Endangered Species Act, Migratory Bird Treaty Act or the Marine Mammal Protection Act and are not targets of fisheries effort. Tag models and attachment procedures varied among species and are described elsewhere (tag models [19] ; attachment methods: blue and humpback whales [30] , [52] ; sea lions and seals [18] , [29] , [53] ; albatrosses and shearwaters [14] , [31] ; leatherback sea turtles [16] ). All animal research was conducted in accordance with Institutional Animal Care and Use Committee protocols from Stanford University and the University of California. Tracking data were collected via the Argos satellite system [54] for marine mammals, Laysan albatrosses and leatherback sea turtles, and via archival tags that determined geolocations via ambient light levels for sooty shearwaters and post-breeding black-footed albatrosses [14] , [32] , [55] . All Argos tracks were processed using a state-space model [56] to handle observation error from Argos (whales [30] , California sea lions [57] , elephant seals [58] and leatherback sea turtles [16] ) except Laysan albatrosses, which were processed using speed and distance filters (details in ref. 32 ). Geolocation tracks were processed following methods described in refs 59 , 55 resulting in two locations per day. Tracks were interpolated to 1-h intervals using hermite (whales, pinnipeds and turtles) or Bezier (seabirds) splines following ref. 60 to approximate animal locations between reported positions. To determine the relative use of marine habitat by animal species, we constructed gridded animal UDs (the probability of an animal being found in a given cell [27] ) for the entire range of each species distribution using 0.25° × 0.25° cells [43] . Before constructing UDs, we normalized tracks of non-central place foragers (whales and turtles) to account for tracks of different durations. We weighted each location by the inverse number of individuals with locations on that same day for each species, using an 85th percentile threshold beyond which all locations received the same weight as the threshold day [19] . When using tracking data, some tagging bias is inevitable as tagging is carried out where logistically feasible, which is largely determined by where animals are commonly found. All of these predators, however, are widely ranging and carried tags for many months to years, and tagging has greatly increased our understanding of animal distributions [21] . Further, null model simulations on this data set have shown that movement of predators is robust to tagging location and that predator ‘hotspots,’ congregations or areas of intense use are behaviourally driven and real, and not simply an artifact of tagging locations [19] . At minimum, our results are conservative in that although the aggregations we identified are real and representative, there may be other regions that might be identified with a larger or more dispersed tagging effort. Determining CUI scores Previous studies of cumulative human impacts have used publicly available ecosystem impact and stressor intensity data [12] to estimate impacts on species [11] , [15] , [24] . The nature of anthropogenic impacts on ecosystems is different from impacts on marine predators; thus, we created new cumulative impact scores for stressors specific to each marine predator species, accounting for unique vulnerabilities of each species to each stressor. We calculated the CUI score for all species combined and on each of the three species groups (marine mammals, seabirds and leatherback sea turtles) for each 0.25° × 0.25° cell as: where D i is the normalized and log-transformed value of intensity of an anthropogenic stressor at location i , S j is the probability distribution of species j being present in a given cell and u i,j is the impact weight for anthropogenic impact i for species j , similar to ref. 38 . The intensity of an anthropogenic stressor was estimated using the driver or stressor data created at 1 km 2 resolution as part of Halpern et al. [38] Twenty-four drivers and stressors associated with climate, coastlines, fishing, pollution and shipping were included in the analysis and spatial driver and stressor data were scaled up or down to 0.25° × 0.25° cells, depending on the resolution of the driver or stressor data ( Supplementary Table S1 ; see ref. 38 for a detailed description of data layers). Both the median and maximum stressor values for each cell were examined and each produced similar CUI patterns; the maximum value for the stressor data for each 0.25° cell was used for subsequent analyses to capture maximum potential impacts. The vulnerability weights of each driver or stressor ( u i,j ) were determined via a literature review to determine expected impacts for each of the eight species; summaries are detailed in Supplementary Note 1 . The vulnerability weight of each stressor was determined through ranking of six measures: (1) stressor frequency, (2) if the impact was direct or indirect, (3) resistance of the species to the stressor, (4) recovery time of an individual from the impact, (5) relative impact on reproduction and (6) relative impact on the population (detailed description in Supplementary Table S4 ). All vulnerability measures were normalized (scaled between 0 and 1) and summed to obtain a weight for each stressor for each species ( Supplementary Table S2 ; Supplementary Note 1 for summary of each impact). Weights for each stressor were multiplied by the normalized, log-transformed value of intensity of the corresponding stressor within each cell to determine its predicted impact. The level of a species’ use of a cell ( S j ) was obtained from the UDs described above and summed across species within each cell for each species group. To create the overall CUI score, the summed impact scores were multiplied by the summed UD for each cell. Metric and species group comparisons We evaluated potential differences in the intensity of animal use, cumulative impacts and CUIs of all species combined, within each species group and among species groups in relation to the continental shelf and the sanctuaries. For combined species and within-species group comparisons, we determined the mean and s.d. of UDs, cumulative impacts (that is, stressor data weighted by species vulnerability but without animal distributions included) and CUIs for each species group on and off the continental shelf (defined as depths greater than 200 m) and inside versus outside the sanctuary boundaries. We chose these spatial regions to reflect different management strategies and because impacts have been shown to be different on versus off the continental shelves [38] , [39] . We performed two-tailed Welch’s t -tests assuming unequal variances within each species group to determine if animal use, cumulative impacts and CUIs were different in relation to the continental shelf and the sanctuaries. UD and CUI data were first log transformed to meet normality assumptions. For among species group comparisons, we compared the mean UDs, cumulative impacts and CUIs among species groups. Analyses of percentage on/off the continental shelf and inside/outside the sanctuaries were conducted separately (that is, four separate comparisons) using one-factor ANOVAs and Tukey’s HSD tests to determine differences in intensity of animal use, cumulative impacts and CUIs of the groups using the log-transformed UD and CUI data. Spatial distribution of metrics and species groups We determined the distribution of ‘core’ animal use, cumulative impact and CUI cells to highlight where species and impacts were greatest in relation to the continental shelf and the sanctuaries, and where mitigation efforts could potentially have maximum impact. The core was defined as the values equivalent to the 50% or greater quartiles for UDs, cumulative impacts and CUIs. We first normalized by the number of cells found on and off the shelf and inside and outside the sanctuaries. Influence of CUI layers To determine the influence of the individual CUI layers (for example, ultraviolet radiation CUI across species groups) on the overall CUI, we calculated the mean, variance and maximum contribution values across each cell for each CUI layer within each of the species groups and all species combined. We used pairwise linear regressions to determine how well each individual CUI layer was able to predict the pattern of the overall CUI [38] . These were used to determine which stressors had the greatest effect on the species groups and to identify which justify the most mitigation effort. Finally, to understand the spatial distribution of different cumulative impacts, cumulative impact layers were grouped based on their similarity or means of mitigation (for example, climate, coastal, fishing, pollution and shipping; Supplementary Table S1 ). Stressors classified as having a direct impact on species were also grouped together ( Supplementary Table S2 ). These groupings were intended to capture the management responsibilities of specific agencies or groups of agencies or related mitigation techniques. How to cite this article: Maxwell, S. M. et al. Cumulative human impacts on marine predators. Nat. Commun. 4:2688 doi: 10.1038/ncomms3688 (2013).